Two distinct secretion systems facilitate tissue invasion by the rice blast fungusMagnaporthe oryzae To cause plant diseases, pathogenic micro-organisms secrete effector proteins into host tissue to suppress immunity and support pathogen growth. Bacterial pathogens have evolved several distinct secretion systems to target effector proteins, but whether fungi, which cause the major diseases of most crop species, also require different secretory mechanisms is not known. Here we report that the rice blast fungus Magnaporthe oryzae possesses two distinct secretion systems to target effectors during plant infection. Cytoplasmic effectors, which are delivered into host cells, preferentially accumulate in the biotrophic interfacial complex, a novel plant membrane-rich structure associated with invasive hyphae. We show that the biotrophic interfacial complex is associated with a novel form of secretion involving exocyst components and the Sso1 t -SNARE. By contrast, effectors that are secreted from invasive hyphae into the extracellular compartment follow the conventional secretory pathway. We conclude that the blast fungus has evolved distinct secretion systems to facilitate tissue invasion. Biotrophic pathogens grow in intimate contact with living host cells and deliver effector proteins into and around these host cells [1] , [2] , [3] , [4] . In pathogenic bacteria, effectors serve a variety of functions, including induction of host cell entry by intracellular pathogens, modulation of host cell signalling and suppression of immune responses. These distinct functions are associated with specific forms of secretion that operate during pathogenesis [5] , [6] . Eukaryotic microbial pathogens, such as fungi and oomycetes, possess even larger numbers of effector proteins that are secreted during host infection [3] , [4] , [7] , [8] . They serve to suppress immunity [9] , [10] , [11] , modulate metabolism [12] and prevent recognition of the invading microbe [13] , [14] . Although the functions of most of these effectors are still unknown, it is increasingly clear that fungal effectors are delivered both to the inside of host cells, as well as to the host–pathogen interface during infection. The ascomycete fungus Magnaporthe oryzae causes rice blast, the most serious disease of cultivated rice and a major threat to global food security [15] , [16] , [17] . Additionally, a wheat-adapted population of M. oryzae has recently emerged to cause wheat blast disease in South America, and this fungus now also poses a threat to global wheat production [18] , [19] . To cause disease, the fungus uses a special infection cell called an appressorium, which ruptures the rice cuticle and allows the fungus entry into the epidermal cells [16] , [20] , [21] . M. oryzae then invades rice tissue using specialized filamentous invasive hyphae (IH), which successively occupy living rice cells [22] and colonize tissue extensively before the appearance of disease symptoms. Host cells are initially invaded by narrow tubular primary hyphae that subsequently develop into enlarged, bulbous IH ( Fig. 1a ) [22] . Morphologically, bulbous IH are constricted at septal junctions, resembling pseudohyphae produced by the human fungal pathogen Candida albicans [23] , [24] . Differentiation to a specialized invasive hypha recurs for each new filamentous hypha that enters a living host cell ( Fig. 1a ), and this differentiation process appears critical for disease development. 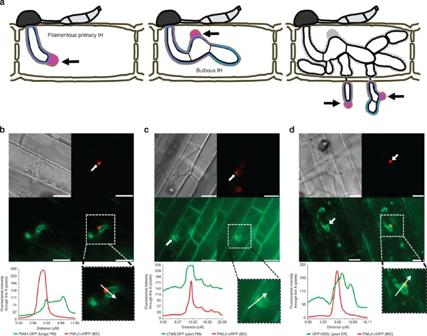Figure 1: The biotrophic interfacial complex is a plant-derived membrane-rich structure. (a) Schematic representation of the differentiation of a filamentous primary invasive hypha (left, ~22–25 h post inoculation, h.p.i.) into a pseudohyphal-like bulbous invasive hypha (middle, ~26–30 h.p.i.) in a first-invaded rice cell. This differentiation occurs for each new hypha invading a living neighbour cell (right, ~36–40 h.p.i.). Cytoplasmic effectors show preferential accumulation in the BIC (black arrows), which is first located in front of the growing primary hyphal tips, and then remains behind beside the first-differentiated bulbous IH cell. Typical accumulation patterns for cytoplasmic (magenta) and apoplastic (blue) effectors are shown within the EIHM (tan) compartment enclosing the IH. The EIHM appears to lose integrity when the fungus has moved into neighbour cells (dotted line). (b–d) Live cell imaging ofM. oryzaeinfection of rice sheath epidermal cells with the BIC (red) visualized by accumulation of IH-secreted Pwl2:mRFP. Clockwise, images are DIC; mRFP (white arrow indicates BIC); merged GFP (green) and mRFP (red); and GFP alone. Below, white arrow in the inset shows the path for fluorescence intensity distribution linescans on the left. (b) The BIC (red) is located outside the fungal plasma membrane (green), which was visualized by expression ofM. oryzaeATPase Pma1:GFP, here imaged at 23 h.p.i. Lack of co-localization between Pwl2:mRFP and Pma1:GFP, indicated by separate subcellular distribution maxima, confirms that the BIC does not contain fungal plasma membrane. (c) The BIC (red) co-localized with intense fluorescence from a rice plasma membrane marker LTi6B:GFP (green), visualized after infection of transgenic rice (at 24 h.p.i.). Note that the plant plasma membrane marker also outlined the entire IH, consistent with invagination around the fungus during cell invasion. Co-localization of fluorescence intensity maxima indicates that the BIC contains material derived from plant plasma membrane. (d) The BIC (red) co-localized with fluorescence from rice ER marker GFP:HDEL (green) expressed in transgenic plants and imaged at 24 h.p.i. Fluorescence intensity maxima demonstrate plant ER localized with and closely surrounding the BIC. White asterisks indicate appressoria. Scale bars, 10 μm. Figure 1: The biotrophic interfacial complex is a plant-derived membrane-rich structure. ( a ) Schematic representation of the differentiation of a filamentous primary invasive hypha (left, ~22–25 h post inoculation, h.p.i.) into a pseudohyphal-like bulbous invasive hypha (middle, ~26–30 h.p.i.) in a first-invaded rice cell. This differentiation occurs for each new hypha invading a living neighbour cell (right, ~36–40 h.p.i.). Cytoplasmic effectors show preferential accumulation in the BIC (black arrows), which is first located in front of the growing primary hyphal tips, and then remains behind beside the first-differentiated bulbous IH cell. Typical accumulation patterns for cytoplasmic (magenta) and apoplastic (blue) effectors are shown within the EIHM (tan) compartment enclosing the IH. The EIHM appears to lose integrity when the fungus has moved into neighbour cells (dotted line). ( b – d ) Live cell imaging of M. oryzae infection of rice sheath epidermal cells with the BIC (red) visualized by accumulation of IH-secreted Pwl2:mRFP. Clockwise, images are DIC; mRFP (white arrow indicates BIC); merged GFP (green) and mRFP (red); and GFP alone. Below, white arrow in the inset shows the path for fluorescence intensity distribution linescans on the left. ( b ) The BIC (red) is located outside the fungal plasma membrane (green), which was visualized by expression of M. oryzae ATPase Pma1:GFP, here imaged at 23 h.p.i. Lack of co-localization between Pwl2:mRFP and Pma1:GFP, indicated by separate subcellular distribution maxima, confirms that the BIC does not contain fungal plasma membrane. ( c ) The BIC (red) co-localized with intense fluorescence from a rice plasma membrane marker LTi6B:GFP (green), visualized after infection of transgenic rice (at 24 h.p.i.). Note that the plant plasma membrane marker also outlined the entire IH, consistent with invagination around the fungus during cell invasion. Co-localization of fluorescence intensity maxima indicates that the BIC contains material derived from plant plasma membrane. ( d ) The BIC (red) co-localized with fluorescence from rice ER marker GFP:HDEL (green) expressed in transgenic plants and imaged at 24 h.p.i. Fluorescence intensity maxima demonstrate plant ER localized with and closely surrounding the BIC. White asterisks indicate appressoria. Scale bars, 10 μm. Full size image During biotrophic invasion, M. oryzae expresses many low-molecular-weight biotrophy-associated secreted (Bas) proteins, including known effector proteins, and these proteins possess classical signal peptides, which facilitate delivery into the endoplasmic reticulum (ER) [8] , [25] , [26] . The ER chaperone Lhs1 is furthermore required for secretion of effectors [27] . Previous in planta analyses have involved live-cell imaging of M. oryzae strains secreting chimeric effector proteins labelled with carboxy-terminal green fluorescent protein (GFP), monomeric red fluorescent protein (mRFP) or monomeric Cherry (mCherry). Secreted effectors show distinct patterns of accumulation within the extra-invasive hyphal membrane (EIHM) compartment enclosing IH growing in rice cells [14] , [25] , [28] . Apoplastic effectors, which do not enter host cells, are generally dispersed and retained within the EIHM compartment, where they outline the entire IH. By contrast, cytoplasmic effectors preferentially accumulate in the biotrophic interfacial complex (BIC) [28] , a membrane-rich structure that initially appears adjacent to primary hyphal tips, but is later positioned subapically as IH develop within rice cells ( Fig. 1a ). Fluorescent effector proteins that accumulate in BICs appear to be translocated across the EIHM into the cytoplasm of living rice cells [28] . Translocation of effectors into rice cells has been most clearly visualized by expression of fluorescent effector fusion proteins with an artificially added C-terminal nuclear localization signal (NLS). The NLS serves to enhance the sensitivity of effector detection in host cells by concentrating them in the rice nucleus. Using this sensitive assay, it has been shown that some translocated cytoplasmic effectors move ahead of the invading pathogen, into three to four layers of surrounding rice cells, presumably to prepare these cells for fungal colonization [28] . The distinct localization patterns of cytoplasmic and apoplastic effectors within the EIHM compartment raise questions regarding the mechanism by which effectors are secreted by IH within living plant cells. Protein secretion associated with apical tip growth in filamentous fungi involves the Spitzenkörper, the vesicle supply centre feeding vesicles to growing hyphal tips [29] , [30] , [31] , [32] . The three-component polarisome complex nucleates actin cables for transporting vesicles to the growth point. Near the polarized secretion site, vesicles dock with the exocyst, a complex of eight proteins that has been implicated in tethering vesicles to the target membrane before fusion. However, it is becoming clear that the exocyst has a role at many sites in a cell as a spatiotemporal regulator of membrane trafficking in response to diverse signals [33] . Fusion of secretory vesicles to the plasma membrane is then directed by SNAREs (soluble N -ethylmaleimide-sensitive factor attachment protein receptors), involving a v-SNARE on the vesicle and a t-SNARE on the membrane. Hyphal growth and secretion in filamentous fungi was thought to occur exclusively at the hyphal tips, but this no longer appears to be the case [29] . In Trichoderma reesei and Aspergillus oryzae , exocytosis mediated by SNARE proteins can also occur in subapical hyphal compartments [34] , [35] . In this study, we focus on investigating how the fungus secretes effectors during host cell invasion. We were specifically interested in determining whether effectors destined for translocation to host cells follow the same secretory route as those that accumulate in the apoplast. We present evidence for two distinct secretory pathways in M. oryzae . We show that BICs are plant-derived, membrane-rich interfacial structures associated with accumulation of effectors that ultimately enter host cells, and that subapical BIC-associated IH cells are enriched in secretion machinery components. Using a combination of pharmacological and gene functional analyses, we show that the conventional fungal ER-Golgi secretion pathway is involved in secretion of apoplastic effectors, but not cytoplasmic effectors, and conversely, that cytoplasmic effectors require exocyst components Exo70 and Sec5 for efficient secretion. Taken together, our results are consistent with operation of two distinct secretory pathways for effector delivery during plant infection by the rice blast fungus. The biotrophic interfacial complex is a plant-derived structure To define the location and structure of the BIC, we first generated fungal transformants expressing fluorescently labelled plasma membrane ( Fig. 1b ) and cytoplasmic ( Supplementary Fig. S1 ) markers, together with BIC-localized cytoplasmic effectors such as Pwl2, which prevents pathogenicity towards weeping lovegrass ( Eragrostis curvula ) [36] . The fungal plasma membrane was visualized by expression of the M. oryzae membrane ATPase Pma1 as a translational fusion to GFP ( Fig. 1b ). During growth inside rice cells, fungal transformants expressing Pma1:GFP and Pwl2:mRFP consistently showed red fluorescence of BIC-localized Pwl2:mRFP outside the green fluorescence in the labelled fungal plasma membrane, confirming that the BIC lies outside the fungal plasma membrane. We then generated transgenic rice lines expressing the fluorescently labelled plasma membrane marker Lti6B-GFP and the ER marker HDEL-GFP. Imaging of fungus expressing Pwl2:mRFP invading these fluorescently labelled rice lines provided evidence that BICs are associated with concentrated regions of plant plasma membrane and ER ( Fig. 1c ). When considered together, these results demonstrate that the BIC is a plant-derived interfacial structure and that effectors must be secreted by the invading fungus in order to be observed so specifically at the BIC. Organization of secretory complexes within invasive hyphae of M. oryzae To investigate the mechanisms of effector secretion by IH inside rice cells, we identified M. oryzae orthologues of genes implicated in polarized growth and secretion ( Supplementary Fig. S2 and Supplementary Table S1 ) [23] , [30] , [32] , [33] . These genes encoded the myosin motor regulatory component Mlc1 (MGG_09470.6) (associated with the Spitzenkörper in C. albicans [23] ), polarisome component Spa2 (MGG_03703.6) and exocyst component Exo70 (MGG_01760.6). We also identified genes encoding v-SNARE Snc1 (MGG_12614.6) and t-SNARE Sso1 (MGG_04090.6), which together mediate docking and fusion of vesicles with the plasma membrane target site [35] . All genes were expressed in M. oryzae under control of their native promoters and with C-terminal translational fusions of GFP, except for Snc1, which was expressed with an amino-terminal fusion of GFP. Each putative secretion component localized with fluorescence concentrated at the tips of vegetative hyphae growing on agar medium, as expected ( Fig. 2 ). Spitzenkörper localization of Mlc1:GFP was confirmed by co-localization with the Styryl dye FM4-64, the endocytotic tracer dye that is a generally accepted Spitzenkörper marker ( Fig. 2a ) [23] , [37] , [38] , [39] . These secretory components also concentrated in the growing tips of primary hyphae adjacent to BICs ( Figs 2c and 3a ). Therefore, secretory machineries of vegetative and primary IH appear to be similarly organized. 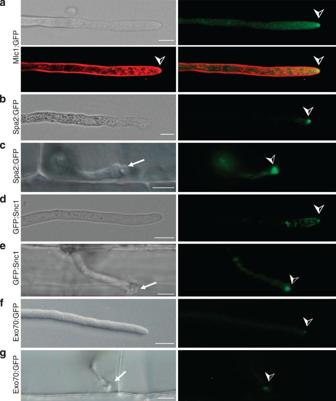Figure 2: Secretion components localize similarly in vegetative and primary hyphae. Fluorescent secretory components () were imaged inM. oryzaefilamentous vegetative hyphaein vitro(a,b,d,f) and in tubular primary hyphae growing in rice cells (c,e,g). BICs (white arrows) were observed adjacent to the primary hyphal tips even without fluorescent labelling. (a) Spitzenkörper marker Mlc1:GFP (green) co-localizes (yellow) with the endocytic tracker dye FM4-64 (red) at tips of vegetative hyphae. This confocal image was acquired 10 min after FM4-64 addition. Images clockwise from upper left are bright-field; GFP; merged GFP and FM4-64; and FM4-64 alone. Similarly, Mlc1:GFP identifies Spitzenkörper in primary hyphae inside rice cells (Fig. 3a). (b–g) Images from left to right are bright-field; and GFP alone. (b) Polarisome component Spa2:GFP localizes to the tip of a vegetative hypha. (c) Polarisome component Spa2:GFP concentrates at the primary hyphal tip behind the BIC at 22 h.p.i. (d) v-SNARE GFP:Snc1 localizes at the vegetative hyphal tip. (e) v-SNARE GFP:Snc1 localizes in a bright fluorescent punctum near the primary hyphal tip at 24 h.p.i. (f) Exocyst component Exo70:GFP localizes at the vegetative hyphal tip. (g) Exocyst component Exo70:GFP localizes at the primary hyphal tip at 24 h.p.i. Scale bars, 5 μm. Figure 2: Secretion components localize similarly in vegetative and primary hyphae. Fluorescent secretory components ( ) were imaged in M. oryzae filamentous vegetative hyphae in vitro ( a , b , d , f ) and in tubular primary hyphae growing in rice cells ( c , e , g ). BICs (white arrows) were observed adjacent to the primary hyphal tips even without fluorescent labelling. ( a ) Spitzenkörper marker Mlc1:GFP (green) co-localizes (yellow) with the endocytic tracker dye FM4-64 (red) at tips of vegetative hyphae. This confocal image was acquired 10 min after FM4-64 addition. Images clockwise from upper left are bright-field; GFP; merged GFP and FM4-64; and FM4-64 alone. Similarly, Mlc1:GFP identifies Spitzenkörper in primary hyphae inside rice cells ( Fig. 3a ). ( b – g ) Images from left to right are bright-field; and GFP alone. ( b ) Polarisome component Spa2:GFP localizes to the tip of a vegetative hypha. ( c ) Polarisome component Spa2:GFP concentrates at the primary hyphal tip behind the BIC at 22 h.p.i. ( d ) v-SNARE GFP:Snc1 localizes at the vegetative hyphal tip. ( e ) v-SNARE GFP:Snc1 localizes in a bright fluorescent punctum near the primary hyphal tip at 24 h.p.i. ( f ) Exocyst component Exo70:GFP localizes at the vegetative hyphal tip. ( g ) Exocyst component Exo70:GFP localizes at the primary hyphal tip at 24 h.p.i. Scale bars, 5 μm. 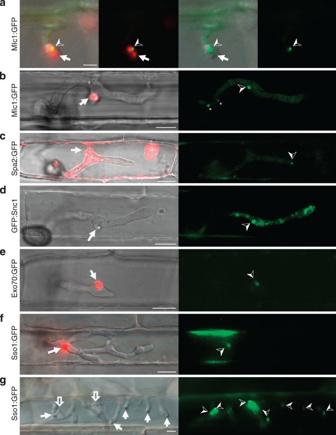Figure 3: BIC-associated IH cells contain components of the secretory machinery. All images are representative of at least five biological replicates with >50 images each. BICs are labelled by arrows in all panels and by red fluorescence from Pwl2:mRFP in all panels exceptdandg. Unless mentioned otherwise, images left to right are: merged bright-field and mRFP (red); and GFP alone (green). (a) The myosin regulatory light chain Mlc1:GFP () labels the Spitzenkörper at the primary hyphal tip before hyphal differentiation at 24 h.p.i. Images left to right: merged bright-field, GFP and mRFP; merged GFP and mRFP; merged bright-field and GFP; and GFP alone. Scale bar, 5 μm. (b) After differentiation of bulbous IH at 27 h.p.i., Mlc1:GFP accumulates in a large fluorescent punctum in the BIC-associated bulbous IH cell () and near septa (*). Spitzenkörper-like fluorescence is not observed in growing bulbous IH tips. (c) Polarisome component Spa2:GFP localizes as a distinct punctum at the tip of growing IH () at 27 h.p.i. Spa2 fluorescence is not observed in the subapical BIC-associated IH cell. In this image, saturated fluorescence from Pwl2:mRFP labels the rice cytoplasm and nucleus (*). This saturated Pwl2:mRFP fluorescence is seen in the EIHM compartment surrounding the BIC-associated cells, as previously reported28. (d) v-SNARE GFP:Snc1 localizes to a large fluorescent punctum () in the BIC-associated IH cell and to smaller vesicles in growing IH at 27 h.p.i. Images left to right: bright-field; and GFP alone. (e) Faint fluorescence from exocyst component Exo70:GFP can be observed in the subapical BIC-associated cell at 28 h.p.i. (f) t-SNARE Sso1:GFP () localizes in the BIC-associated IH cell near the BIC in a first-invaded rice cell at 27 h.p.i. (g) t-SNARE Sso1:GFP () in a second-invaded cell accumulated near BICs, as crescents at the tips of five primary IH (white arrows), and as puncta in two BIC-associated IH cells after differentiation (outline arrows). Shown at 40 h.p.i. (as described inFig. 1a, right panel). Images left to right: bright-field; and GFP alone. Scale bars, 10 μm unless stated otherwise. Full size image Figure 3: BIC-associated IH cells contain components of the secretory machinery. All images are representative of at least five biological replicates with >50 images each. BICs are labelled by arrows in all panels and by red fluorescence from Pwl2:mRFP in all panels except d and g . Unless mentioned otherwise, images left to right are: merged bright-field and mRFP (red); and GFP alone (green). ( a ) The myosin regulatory light chain Mlc1:GFP ( ) labels the Spitzenkörper at the primary hyphal tip before hyphal differentiation at 24 h.p.i. Images left to right: merged bright-field, GFP and mRFP; merged GFP and mRFP; merged bright-field and GFP; and GFP alone. Scale bar, 5 μm. ( b ) After differentiation of bulbous IH at 27 h.p.i., Mlc1:GFP accumulates in a large fluorescent punctum in the BIC-associated bulbous IH cell ( ) and near septa (*). Spitzenkörper-like fluorescence is not observed in growing bulbous IH tips. ( c ) Polarisome component Spa2:GFP localizes as a distinct punctum at the tip of growing IH ( ) at 27 h.p.i. Spa2 fluorescence is not observed in the subapical BIC-associated IH cell. In this image, saturated fluorescence from Pwl2:mRFP labels the rice cytoplasm and nucleus (*). This saturated Pwl2:mRFP fluorescence is seen in the EIHM compartment surrounding the BIC-associated cells, as previously reported [28] . ( d ) v-SNARE GFP:Snc1 localizes to a large fluorescent punctum ( ) in the BIC-associated IH cell and to smaller vesicles in growing IH at 27 h.p.i. Images left to right: bright-field; and GFP alone. ( e ) Faint fluorescence from exocyst component Exo70:GFP can be observed in the subapical BIC-associated cell at 28 h.p.i. ( f ) t-SNARE Sso1:GFP ( ) localizes in the BIC-associated IH cell near the BIC in a first-invaded rice cell at 27 h.p.i. ( g ) t-SNARE Sso1:GFP ( ) in a second-invaded cell accumulated near BICs, as crescents at the tips of five primary IH (white arrows), and as puncta in two BIC-associated IH cells after differentiation (outline arrows). Shown at 40 h.p.i. (as described in Fig. 1a , right panel). Images left to right: bright-field; and GFP alone. Scale bars, 10 μm unless stated otherwise. Full size image Although Mlc1:GFP identified Spitzenkörper at primary hyphal tips in planta ( Fig. 3a ), Spitzenkörper were not observed at the hyphal growth points after differentiation of bulbous IH ( Fig. 3b ). This result is consistent with loss of the ball-like Spitzenkörper after differentiation of C. albicans hyphae into pseudohyphae [23] . In bulbous IH, Mlc1:GFP identified a fluorescent spot near each septum as well as a single larger fluorescent spot in the subapical BIC-associated cell, which was no longer growing ( Fig. 3b ). In contrast, polarisome marker Spa2:GFP remained localized at hyphal growth points ( Fig. 3c ), and was not observed in BIC-associated IH cells. Similarly to Mlc1:GFP, the SNARE proteins GFP:Snc1 and Sso1:GFP and exocyst protein Exo70:GFP each showed significant focal fluorescence in subapical BIC-associated cells in addition to fluorescence elsewhere in the hyphae ( Fig. 3d–f ). For example, GFP:Snc1 also localized as smaller vesicles, especially at hyphal growth points ( Fig. 3d ). In subsequently invaded cells, all markers first showed significant fluorescence at tips of the initially tubular hyphae that entered each rice cell. After differentiation to bulbous IH, all markers except Spa2:GFP showed significant localization in subapical BIC-associated IH cells. This is shown for Sso1:GFP fluorescence in the seven visible hyphae growing in a second-invaded cell ( Fig. 3g ). We conclude that filamentous primary hyphae and pseudohyphal-like bulbous IH are distinct morphological cell types and that switching between tubular and bulbous IH in planta may involve a spatiotemporal reorientation of secretory machinery. Additionally, after differentiation and further growth, we conclude that subapical bulbous IH cells associated with BICs are capable of active secretion. Brefeldin A treatment identifies distinct effector secretion pathways To test the nature of fungal secretion, we first exposed M. oryzae IH to Brefeldin A (BFA), which inhibits conventional ER-to-Golgi secretion in fungi [40] . For these experiments, we used a M. oryzae strain expressing both apoplastic effector Bas4:GFP [25] and cytoplasmic effector Pwl2:mCherry:NLS ( Fig. 4a ). We found that the apoplastic effector Bas4:GFP was retained in the hyphal ER within 3 h of exposure of infected rice tissue to BFA, but cytoplasmic effector Pwl2:mCherry:NLS still exhibited BIC accumulation with no observable fluorescence inside the hyphal ER, even with longer periods of exposure ( Fig. 4b ). The distinct BFA localization patterns for Pwl2 and Bas4 were independent of the fluorescent proteins used and the added NLS, indicating that effector sequences controlled the distinct secretion properties ( Supplementary Fig. S3a ). To determine whether these effects were general, we tested additional cytoplasmic effectors AVR-Pita (ref. 8 ) ( Fig. 4c ), Bas1 (ref. 25 ) ( Fig. 4c ) and Bas107 ( Supplementary Fig. S3b ). Secretion and BIC localization of all three continued in the presence of BFA with no visible accumulation of fluorescence inside IH. By contrast, secretion of additional apoplastic effectors Slp1:GFP [14] and Bas113:mRFP was blocked by BFA treatment ( Supplementary Fig. S3c ). 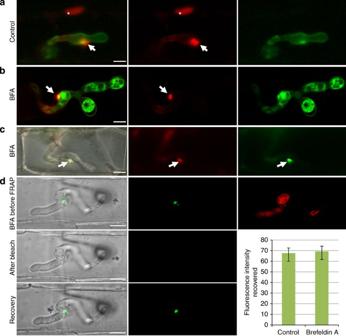Figure 4: Brefeldin A blocks secretion of apoplastic but not of cytoplasmic effectors. (a–c) Images left to right: either merged bright-field, mCherry and GFP or merged mCherry and GFP; mCherry alone; and GFP alone. (a) After secretion, cytoplasmic effector Pwl2:mCherry:NLS (red) shows preferential BIC localization (arrow) and translocation into the rice cell, where it accumulates in the rice nucleus (*). Bas4:GFP shows apoplastic localization outlining the IH. (b) In the presence of BFA, Pwl2:mCherry:NLS remains BIC-localized (arrow), but Bas4:GFP (green) is retained in the fungal ER, imaged with the same transformant in (a) 10 h after exposure to BFA. (c) Cytoplasmic effectors Bas1:mRFP (red, middle) and AVR-Pita:GFP (green, right) still co-localized in the BIC (arrow) after 5 h exposure to BFA. (d) Fluorescence recovery after photobleaching (FRAP) demonstrates continuous secretion of Pwl2:GFP into the BIC in the presence of BFA. Rice tissue infected by a fungal strain expressing Pwl2:GFP and Bas4:mRFP was incubated in BFA for 3 h before photobleaching of Pwl2:GFP in the BIC. Secretion of Bas4:mRFP had been blocked at this point. FRAP results were identical in the presence or absence of BFA (P=0.019). Bars show mean fluorescence intensity recovery after bleaching (mean±s.d., four FRAP experiments). Images left to right before photobleaching: merged bright-field and GFP; GFP alone; and mRFP alone. Images left to right after photobleaching and recovery: merged bright-field and GFP; and GFP alone. Scale bars, 10 μm. Figure 4: Brefeldin A blocks secretion of apoplastic but not of cytoplasmic effectors. ( a – c ) Images left to right: either merged bright-field, mCherry and GFP or merged mCherry and GFP; mCherry alone; and GFP alone. ( a ) After secretion, cytoplasmic effector Pwl2:mCherry:NLS (red) shows preferential BIC localization (arrow) and translocation into the rice cell, where it accumulates in the rice nucleus (*). Bas4:GFP shows apoplastic localization outlining the IH. ( b ) In the presence of BFA, Pwl2:mCherry:NLS remains BIC-localized (arrow), but Bas4:GFP (green) is retained in the fungal ER, imaged with the same transformant in ( a ) 10 h after exposure to BFA. ( c ) Cytoplasmic effectors Bas1:mRFP (red, middle) and AVR-Pita:GFP (green, right) still co-localized in the BIC (arrow) after 5 h exposure to BFA. ( d ) Fluorescence recovery after photobleaching (FRAP) demonstrates continuous secretion of Pwl2:GFP into the BIC in the presence of BFA. Rice tissue infected by a fungal strain expressing Pwl2:GFP and Bas4:mRFP was incubated in BFA for 3 h before photobleaching of Pwl2:GFP in the BIC. Secretion of Bas4:mRFP had been blocked at this point. FRAP results were identical in the presence or absence of BFA ( P =0.019). Bars show mean fluorescence intensity recovery after bleaching (mean±s.d., four FRAP experiments). Images left to right before photobleaching: merged bright-field and GFP; GFP alone; and mRFP alone. Images left to right after photobleaching and recovery: merged bright-field and GFP; and GFP alone. Scale bars, 10 μm. Full size image To confirm that secretion of Pwl2:GFP into BICs continued in the presence of BFA, we performed fluorescence recovery after photobleaching (FRAP) analysis. Using transformants expressing both Pwl2:GFP and Bas4:mRFP, we photobleached Pwl2:GFP in subapical BICs and then monitored fluorescence recovery over time in the presence or absence of BFA. For BFA-treated tissues, retention of Bas4:mRFP in the hyphal ER confirmed that the treatment was effective before fluorescence in the BICs was photobleached. As expected from previous results [28] , full recovery of fluorescence in BICs occurred within 3 h. Identical recovery rates were observed in the presence or absence of BFA ( Fig. 4d ), indicating that the fungus continues to secrete cytoplasmic effector protein into BICs in the presence of BFA. During fungal invasion of rice cells, BFA therefore reproducibly blocked secretion of apoplastic effectors, but not BIC accumulation of cytoplasmic effectors. We tested whether the fungal cytoskeleton is important for effector secretion using the microtubule inhibitor methyl 1-(butylcarbamoyl)-2-benzimidazolecarbamate (MBC) and the actin inhibitor latrunculin A (LatA). Secretion of Bas4:mRFP was impaired when infected rice tissues were treated with MBC or LatA, but secretion of Pwl2:GFP was not visibly impaired ( Supplementary Fig. S4 ). FRAP experiments again confirmed that Pwl2:GFP continued to accumulate in BICs in the presence of MBC or LatA, further supporting the operation of distinct effector secretion mechanisms. Efficient secretion of cytoplasmic effectors requires the exocyst complex We next investigated the protein secretion components necessary for effector secretion. In yeast, Exo70 and Sec5 are subunits of the octameric exocyst complex implicated in spatiotemporal regulation of membrane trafficking [33] . We produced a series of targeted gene replacement mutants for the M. oryzae EXO70 and SEC5 genes in strains expressing fluorescent effectors ( Supplementary Fig. S5 ). These mutants formed normal-appearing IH in first-invaded rice cells. Compared to isogenic wild-type strains imaged in the same experiment ( Fig. 5a ), Δ exo70 and Δ sec5 mutant IH showed significant accumulation of two different cytoplasmic effectors inside BIC-associated cells, indicating that cytoplasmic effector secretion was not efficient in these mutants ( Fig. 5b ). Consistent with impaired effector secretion, we generally observed decreased fluorescence intensity in the BIC and in host nuclei. Secretion of Pwl2:mCherry:NLS was impaired in 60 of 65 randomly imaged infection sites for Δ exo70 mutants ( Fig. 5b ) and in 37 of 40 randomly imaged infection sites for Δ sec5 mutants ( Fig. 5c ). Effector fluorescence inside the IH occurred in the form of small vesicles or vacuole-like puncta. Fluorescence intensity distribution scans confirmed significant retention of cytoplasmic effector fluorescence inside IH cells. Importantly, in ~80% of infection sites with mutant IH, the internal cytoplasmic effector fluorescence was observed in the BIC-associated IH cells and not observed in subsequently formed IH cells. In the remaining infection sites, relatively low levels of Pwl2 fluorescence were observed in some non-BIC-associated IH cells, consistent with low basal levels of expression in these cells at later stages of cell invasion [28] . Similar impaired secretion was observed for independent transformants expressing a different cytoplasmic effector, Bas1:mRFP ( Fig. 5d–f ). That is, fluorescence from Bas1:mRFP was retained inside BIC-associated IH cells in Δ exo70 mutants (in 22 of 28 imaged infection sites) and in Δ sec5 mutants (in 23 of 27 imaged infection sites). Conversely, secretion of the apoplastic effector Bas4 was not impaired in these mutants ( Fig. 5b ). 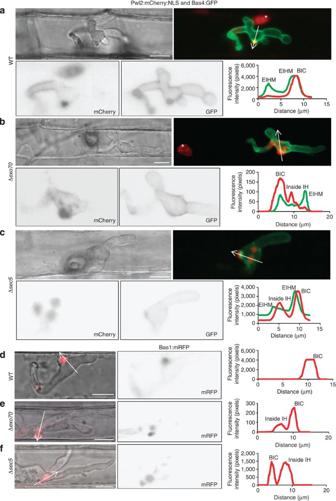Figure 5: Secretion of cytoplasmic effectors involves exocyst components Exo70 and Sec5. (a–c) Wild-type strain Guy11 and corresponding mutants expressed Pwl2:mCherry:NLS and Bas4:GFP. Images clockwise from the upper left: bright-field; merged mCherry (red) and GFP (green); fluorescence intensity linescans for mCherry (red) and GFP (green) along the path of the white arrow; single channel GFP or mCherry fluorescence shown as black and white inverse images, respectively. (a) Pwl2:mCherry:NLS in wild type shows preferential BIC localization, translocation and accumulation in the rice nucleus (white asterisk) with no fluorescence observed in the BIC-associated IH cell. Bas4:GFP localizes to the EIHM compartment. (b) Δexo70mutant shows partial retention of Pwl2:mCherry:NLS, predominantly in the BIC-associated IH cell. Bas4:GFP secretion appears normal. Internal red fluorescence in the BIC-associated IH cell is further visualized by a black and white inverse image (lower left) and by fluorescence intensity scans, which show red fluorescence between the peaks of green fluorescence marking the boundary of the EIHM. Faint red fluorescence in the rice nucleus (white asterisk) is consistent with effector secretion being only partially blocked in the mutants. (c) Δsec5mutant showing partial retention of Pwl2:mCherry:NLS inside the BIC-associated IH cell, but no retention of Bas4:GFP, as further visualized by black and white inverse images and fluorescence intensity scans. (d–f) Images left to right: merged bright-field and mRFP; single channel mRFP fluorescence as a black and white inverse image; and corresponding fluorescence intensity linescan. (d) Wild type Guy11 expressing cytoplasmic effector Bas1:mRFP. Bas1:mRFP fluorescence is not observed inside wild type IH cells. (e) Bas1:mRFP expressed by an Δexo70mutant shows significant retention inside the IH, predominantly in the BIC-associated cells. (f) Bas1:mRFP expressed by an Δsec5mutant strain shows significant retention of Bas1:mRFP inside the IH, predominantly in the BIC-associated cells. Linescans shown are representative of wild type (n=20) and knockout mutants (n=20 for each). Scale bars, 10 μm. Figure 5: Secretion of cytoplasmic effectors involves exocyst components Exo70 and Sec5. ( a – c ) Wild-type strain Guy11 and corresponding mutants expressed Pwl2:mCherry:NLS and Bas4:GFP. Images clockwise from the upper left: bright-field; merged mCherry (red) and GFP (green); fluorescence intensity linescans for mCherry (red) and GFP (green) along the path of the white arrow; single channel GFP or mCherry fluorescence shown as black and white inverse images, respectively. ( a ) Pwl2:mCherry:NLS in wild type shows preferential BIC localization, translocation and accumulation in the rice nucleus (white asterisk) with no fluorescence observed in the BIC-associated IH cell. Bas4:GFP localizes to the EIHM compartment. ( b ) Δ exo70 mutant shows partial retention of Pwl2:mCherry:NLS, predominantly in the BIC-associated IH cell. Bas4:GFP secretion appears normal. Internal red fluorescence in the BIC-associated IH cell is further visualized by a black and white inverse image (lower left) and by fluorescence intensity scans, which show red fluorescence between the peaks of green fluorescence marking the boundary of the EIHM. Faint red fluorescence in the rice nucleus (white asterisk) is consistent with effector secretion being only partially blocked in the mutants. ( c ) Δ sec5 mutant showing partial retention of Pwl2:mCherry:NLS inside the BIC-associated IH cell, but no retention of Bas4:GFP, as further visualized by black and white inverse images and fluorescence intensity scans. ( d – f ) Images left to right: merged bright-field and mRFP; single channel mRFP fluorescence as a black and white inverse image; and corresponding fluorescence intensity linescan. ( d ) Wild type Guy11 expressing cytoplasmic effector Bas1:mRFP. Bas1:mRFP fluorescence is not observed inside wild type IH cells. ( e ) Bas1:mRFP expressed by an Δ exo70 mutant shows significant retention inside the IH, predominantly in the BIC-associated cells. ( f ) Bas1:mRFP expressed by an Δ sec5 mutant strain shows significant retention of Bas1:mRFP inside the IH, predominantly in the BIC-associated cells. Linescans shown are representative of wild type ( n =20) and knockout mutants ( n =20 for each). Scale bars, 10 μm. Full size image Partial retention of these cytoplasmic effectors inside mutant BIC-associated IH cells contrasts with results of extensive imaging of BIC-accumulated effectors in wild-type strains [14] , [25] , [28] , in which fluorescence from cytoplasmic effectors was not observed to be retained inside IH cells. Additionally, Δ exo70 and Δ sec5 mutants showed significant pathogenicity defects on two different rice varieties, when assayed at our independent locations ( Fig. 6a ). This significant loss of pathogenicity would be consistent with these mutants showing inefficient secretion of numerous cytoplasmic effectors with a role in rice blast disease. We conclude that the exocyst is critical both for efficient secretion into BICs and for fungal pathogenicity. 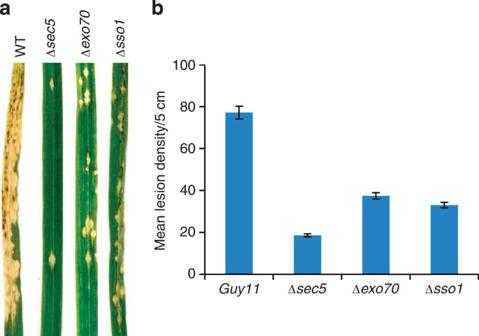Figure 6: Exocyst component and t-SNARE mutants suggest roles in pathogenicity. (a) Targeted deletions of theSEC5,EXO70andSSO1genes in the aggressive Chinese field isolate O-137 (WT) resulted in a significant reduction in pathogenicity on a fully susceptible rice cultivar YT-16 in whole plant spray inoculation assays at Kansas State University. Numbers of lesions formed and lesion sizes were both reduced. (b) Similar pathogenicity defects were observed after inoculation of mutants in the Guy11 (WT) background on rice cultivar CO-39 at the University of Exeter. These data are presented as a bar chart showing the frequency of lesions formed per 5 cm of CO-39 leaf surface (P<0.05 for all mutants;n=30 for each mutant; mean±s.d., three experiments). Figure 6: Exocyst component and t-SNARE mutants suggest roles in pathogenicity. ( a ) Targeted deletions of the SEC5 , EXO70 and SSO1 genes in the aggressive Chinese field isolate O-137 (WT) resulted in a significant reduction in pathogenicity on a fully susceptible rice cultivar YT-16 in whole plant spray inoculation assays at Kansas State University. Numbers of lesions formed and lesion sizes were both reduced. ( b ) Similar pathogenicity defects were observed after inoculation of mutants in the Guy11 (WT) background on rice cultivar CO-39 at the University of Exeter. These data are presented as a bar chart showing the frequency of lesions formed per 5 cm of CO-39 leaf surface ( P <0.05 for all mutants; n =30 for each mutant; mean±s.d., three experiments). Full size image A t-SNARE Sso1 is required for normal BIC development Targeted gene replacement of the M. oryzae t-SNARE SSO1 ( Supplementary Fig. S5 ) produced mutants with both reduced pathogenicity ( Fig. 6a ) and a BIC developmental defect ( Fig. 7a–c ). In contrast to wild-type strains, independent Δ sso1 mutants showed two points of focal accumulation of cytoplasmic effectors. One appeared to be a normal BIC adjacent to the first-differentiated IH cell and the second was a focal fluorescent region adjacent to the primary hypha before the point of differentiation. This ‘double BIC’ phenotype was observed in 32 of 40 random IH expressing Pwl2:mCherry:NLS and in 25 of 30 random IH expressing Bas1:mRFP. This abnormal secretion pattern for cytoplasmic effectors was not observed previously with wild-type strains or mutants defective in other secretion pathway genes. When considered together with the localization pattern of Sso1:GFP ( Fig. 3f ), these results implicate the t-SNARE Sso1 in accumulation of effectors at the BIC. 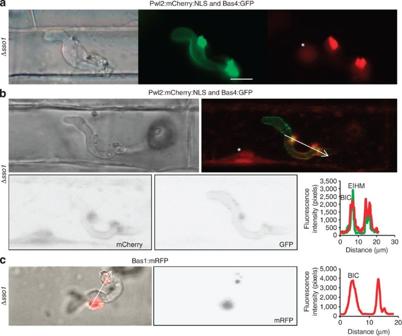Figure 7: t-SNARE mutants suggest a role in BIC development. (a) Δsso1mutant showing inappropriate secretion of Pwl2:mCherry:NLS during plant infection. In addition to BICs in the expected location, second fluorescent foci occurred midway along the primary hyphae. Images left to right: bright-field; GFP (green); and mCherry (red). (b) Another infection site in which Pwl2:mCherry:NLS expressed by an Δsso1mutant strain shows inappropriate secretion. Images clockwise from the upper left: bright-field; merged mCherry (red) and GFP (green); fluorescence intensity linescans for mCherry (red) and GFP (green) along the white arrow; single channel GFP or mCherry fluorescence shown as black and white inverse images. (c) Bas1:mRFP expressed by an Δsso1mutant shows inappropriate secretion. Images left to right: merged bright-field and mRFP; mRFP fluorescence shown as black and white inverse image; and fluorescence intensity linescan along the white arrow. Rice nuclei are indicated by a white asterisk. Linescans shown are representative of wild type (n=20) and knockout mutants (n=20 for each). Scale bars, 10 μm. Figure 7: t-SNARE mutants suggest a role in BIC development. ( a ) Δ sso1 mutant showing inappropriate secretion of Pwl2:mCherry:NLS during plant infection. In addition to BICs in the expected location, second fluorescent foci occurred midway along the primary hyphae. Images left to right: bright-field; GFP (green); and mCherry (red). ( b ) Another infection site in which Pwl2:mCherry:NLS expressed by an Δ sso1 mutant strain shows inappropriate secretion. Images clockwise from the upper left: bright-field; merged mCherry (red) and GFP (green); fluorescence intensity linescans for mCherry (red) and GFP (green) along the white arrow; single channel GFP or mCherry fluorescence shown as black and white inverse images. ( c ) Bas1:mRFP expressed by an Δ sso1 mutant shows inappropriate secretion. Images left to right: merged bright-field and mRFP; mRFP fluorescence shown as black and white inverse image; and fluorescence intensity linescan along the white arrow. Rice nuclei are indicated by a white asterisk. Linescans shown are representative of wild type ( n =20) and knockout mutants ( n =20 for each). Scale bars, 10 μm. Full size image In this report, we have provided evidence that M. oryzae possesses two distinct routes by which it secretes effector proteins during biotrophic invasion of rice ( Fig. 8 ). Apoplastic effectors accumulate extracellularly at the host–pathogen interface and are actively secreted via the conventional secretory process previously defined in filamentous fungi. As expected, this process is inhibited by BFA, implicating Golgi-dependent secretion. By contrast, cytoplasmic effectors destined for delivery inside rice cells are secreted by a different pathway involving the exocyst complex and insensitive to BFA treatment. 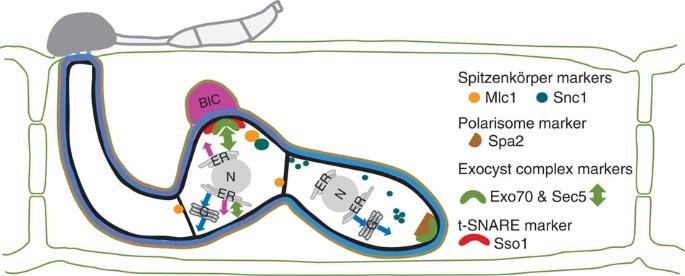Figure 8: Model for effector secretion byM. oryzae. This cartoon shows a bulbous IH at 26–30 h.p.i. inside a rice cell. The EIHM (tan) continues around the BIC. Apoplastic effectors (blue), including Bas4, Bas113 and Slp1, accumulate in the EIHM compartment surrounding the IH, resulting in uniform outlining of the IH. These apoplastic effectors follow the conventional, BFA-sensitive, Golgi-dependent secretion pathway. In contrast, cytoplasmic effectors (magenta), including Pwl2, AVR-Pita, Bas1 and Bas107, accumulate in the BIC beside the first-differentiated bulbous IH cell. To a lesser extent, as observed at saturated fluorescence exposure levels (Fig. 3c), cytoplasmic effectors (magenta dotted line) also accumulate inside the EIHM surrounding the BIC-associated cells (the primary hypha and first-differentiated bulbous IH cell), but they do not outline the subsequently formed bulbous IH cells. These cytoplasmic effectors follow a nonconventional, BFA-insensitive secretion pathway involving exocyst and SNARE proteins. Figure 8: Model for effector secretion by M. oryzae . This cartoon shows a bulbous IH at 26–30 h.p.i. inside a rice cell. The EIHM (tan) continues around the BIC. Apoplastic effectors (blue), including Bas4, Bas113 and Slp1, accumulate in the EIHM compartment surrounding the IH, resulting in uniform outlining of the IH. These apoplastic effectors follow the conventional, BFA-sensitive, Golgi-dependent secretion pathway. In contrast, cytoplasmic effectors (magenta), including Pwl2, AVR-Pita, Bas1 and Bas107, accumulate in the BIC beside the first-differentiated bulbous IH cell. To a lesser extent, as observed at saturated fluorescence exposure levels ( Fig. 3c ), cytoplasmic effectors (magenta dotted line) also accumulate inside the EIHM surrounding the BIC-associated cells (the primary hypha and first-differentiated bulbous IH cell), but they do not outline the subsequently formed bulbous IH cells. These cytoplasmic effectors follow a nonconventional, BFA-insensitive secretion pathway involving exocyst and SNARE proteins. Full size image Previous studies have highlighted the presence of a membrane-rich complex, the BIC, at the host–pathogen interface during rice blast infection [28] . We have now clearly shown that the BIC is a plant-derived interfacial structure that lies outside of the plasma membrane and cell wall of the fungus in a region rich in plant plasma membrane and ER. We have also shown that the fungal exocyst components Exo70 and Sec5 have roles in an unconventional secretory mechanism for blast effectors, which lead to their accumulation at the BIC. Both Δ exo70 and Δ sec5 mutants show inefficient cytoplasmic effector secretion but are still viable inside rice cells, suggesting that there is functional redundancy in the system. Indeed, yeast Exo70 and Sec3 are both exocyst subunits identified as having a role in docking secretory vesicles to active sites of exocytosis [33] . It appears that Exo70 function can be at least partially fulfilled by Sec3 or some unknown component. The exocyst component Sec5 appears to function by interacting with Exo70 and Sec3 to mediate polarized targeting of secretory vesicles to the plasma membrane. Individually, Exo70 and Sec5 are required for efficient secretion of both cytoplasmic effectors we tested. The large pathogenicity defect associated with these mutants could be explained if many cytoplasmic effectors utilize the same unconventional secretion pathway and are inefficiently secreted. The individual IH that we observe in first-invaded cells would fail to thrive during subsequent colonization, and either produce smaller lesions than wild-type IH, or fail to produce macroscopic lesions at all ( Fig. 6 ). Both mutant analysis and localization results indicate that the t-SNARE Sso1 has a role in IH development and effector secretion. The Δ sso1 mutant consistently produces second BIC-like regions of focal effector accumulation midway along the primary hyphae ( Fig. 7 ). This Sso1:GFP localization pattern is consistent with specialized exocytic pathways employing different surface SNAREs at different hyphal sites for cytoplasmic effector secretion and for hyphal growth. There is precedent for the involvement of SNARE proteins in secretion from subapical regions of hyphae. The industrially important cellulolytic filamentous fungus T. reesei has two pathways for exocytosis, which employ different t-SNARE proteins at distinct sites in the hyphae [35] . Secretion of cytoplasmic effectors by a distinct pathway that is predominantly localized to BIC-associated cells is consistent with the BIC being important in effector delivery or sequestration by the host. BICs have been hypothesized as the site of translocation of cytoplasmic effectors into the rice cytoplasm based on a strong correlation between preferential BIC localization of known effectors (such as Pwl2, Avr-Pita and AvrPiz-t) and evidence supporting their translocation to the rice cytoplasm [8] , [11] , [28] . Several aspects of this study are consistent with the idea that BIC-associated bulbous IH cells actively secrete cytoplasmic effectors. First, BIC-associated bulbous IH cells contain concentrated fluorescent foci of GFP-labelled secretory pathway components, the myosin regulatory light chain Mlc1, exocyst component Exo70, v-SNARE Snc1 and t-SNARE Sso1. The only exception to this was the polarisome component Spa2, which we observed only in growing hyphal cells. Retention of Spa2 at bulbous IH growth points after differentiation resembles retention of Spa2 at pseudohyphal growth points after differentiation in C. albicans [23] . Second, fluorescent cytoplasmic effectors accumulate at BICs following photobleaching, and this process is BFA insensitive. Third, cytoplasmic effector proteins accumulate predominantly inside the BIC-associated cells of Δ exo70 and Δ sec5 mutants rather than at hyphal tips, suggesting that they may be secreted predominantly from BIC-associated cells. These results are consistent with new evidence that expression of cytoplasmic effectors is highly upregulated in BIC-associated cells compared to lower basal levels of expression throughout the IH at later infection stages of host cell invasion [28] . We also found that the t-SNARE Sso1 not only localized adjacent to the BIC, but that mutants lacking this gene showed defects in normal BIC development. When considered together, these observations support a central role for the BIC as a destination for secretion of effectors that are ultimately taken up by rice cells. In summary, our results provide evidence that targeting fungal effectors to distinct host compartments may require separate, specialized secretory processes in the rice blast fungus, M. oryzae . Identifying how these processes function will prove pivotal in controlling rice blast disease and also determining the nature and evolution of exocyst processes in fungal pathogens. Live-cell imaging of M. oryzae hyphae Fungal transformants were stored in dried filter papers at −20 °C, and cultured on oatmeal agar plates at 24 °C under continuous light [41] . From fresh fungal cultures, a small plug cut from the hyphal growth zone was placed on the edge of a sterile water agar-coated microscope slide and incubated in a humid chamber for 16–18 h. M. oryzae vegetative hyphae were imaged while growing at a rate of 5–10 μm min −1 on these slides. New fungal transformants were evaluated at 16–18 h post inoculation (h.p.i.) using vegetative hyphae to confirm fluorescence expression. Active growth was documented by time-lapse imaging using AxioVisionLE software, version 4.8. Independent transformants were selected for use based on the highest intensity of the fluorescent marker. These transformants were evaluated during infection in planta by rice sheath inoculations. Rice sheath inoculations were performed as described [22] using the susceptible rice line YT-16. Briefly, 5-cm-long sheath pieces from 3-week-old plants were placed in a glass container under high humidity conditions. Sheaths were placed on acrylic stands to avoid contact with wet paper and to hold epidermal cells directly above the mid-vein horizontally flat for uniform inoculum distribution in the trimmed sheath pieces. A spore suspension (~200 μl of a suspension of 2 × 10 4 spores ml −1 in 0.25% gelatin, Cat. #G-6650, Sigma-Aldrich) was injected into one end of the sheath using a 200-μl pipette. Each segment was trimmed at 22–36 h.p.i. and imaged immediately. Conventional epifluorescence and differential interference contrast microscopy was performed with a Zeiss Axioplan 2 IE MOT microscope, using a × 63 1.2 NA (numerical aperture) C-Apochromat water immersion objective lens. Images were acquired using a Zeiss AxioCam HRc camera and analysed with Zeiss Axiovision digital image-processing software, version 4.8. Fluorescence was observed with an X-Cite®120 (EXFO Life Sciences) mercury lamp source. The filter sets used were: GFP (excitation 480±10 nm, emission 510±10 nm, filter set 41020, Chroma Tech. Corp., Rockingham, VT) and mRFP, mCherry or FM4-64 (excitation 535±25 nm, emission 610±32 1/2 nm, Zeiss). Confocal imaging was performed with a Zeiss Axiovert 200 M microscope equipped with a Zeiss LSM 510 META system using two water immersion objectives, × 40/1.2 NA and × 63/1.2 NA C-Apochromat. Excitation/emission wavelengths were 488 nm/505–550 nm for EGFP, and 543 nm/560–615 nm for mRFP, mCherry and FM4-64. Images were acquired and processed using LSM 510 AIM version 4.2 SP1 software. Identification of M. oryzae secretory pathway genes Sequence data were accessed from the Saccharomyces Genome Database (SGD) ( http://www.yeastgenome.org/sitemap.html ) under the following accession numbers MLC1/YGL106W, SNC1/YAL030W, SPA2/YLL021W, SEC5/YDR166C, SSO1/YPL232W and EXO70/YJL085W. Analysis of the predicted protein sequences was performed using BLASTP [42] from NCBI GeneBank ( http://www.ncbi.nlm.nih.gov/genbank/ ), Broad Institute’s Magnaporthe grisea Genome Database ( http://www.broadinstitute.org/annotation/genome/magnaporthe_grisea/MultiHome.html) , MGOS ( http://www.mgosdb.org/ ), SGD ( http://www.yeastgenome.org/sitemap.html ) and the Biological General Repository for Interaction Datasets (BioGRID) database ( http://www.thebiogrid.org ). Multiple protein sequence alignments were used to find diagnostic patterns to characterize protein families and to detect homology between M. oryzae orthologue sequences and existing families of sequences. These protein sequence alignments were performed using CLUSTALW2 from EMBL-EBI ( http://www.ebi.ac.uk/Tools/clustalw2/index.html ). In ClustalW2 (ref. 43 ), the guide trees, used to guide the multiple alignment, were calculated by a distance matrix method using the Neighbour Joining tree_BLOSUM62 (ref. 44 ). M. oryzae genes selected were MLC1 (MGG_09470), SNC1 (MGG_12614), SPA2 (MGG_03703), EXO70 (MGG_01760), SEC5 (MGG_07150), and SSO1 (MGG_04090). Further details are listed in Supplementary Table S1 . FM4-64 staining and treatment with pharmacological inhibitors Fungal transformants expressing secretion machinery components were treated with FM4-64 (4 μg ml −1 in water). An aqueous 17 mM stock solution of FM4-64 (Cat # 13320, Invitrogen, Carlsbad, CA) was made and stored at −20 °C as described [45] . Vegetative hyphae at ~16–18 h.p.i. on a water agar slide were incubated for 5–30 min in a 10-μM aqueous solution of FM4-64 for uniform staining. In planta , inoculated trimmed leaf sheaths, ~24 h.p.i., were incubated in a 10-μM aqueous working solution for 1–5 h. To examine the effects of brefeldin A (BFA) (Sigma) on IH secretion of effectors in planta , we prepared stock solutions of BFA, 10 mg ml −1 , in dimethyl sulphoxide (DMSO, Sigma) according to Bourett and Howard [46] . We incubated the leaf sheath tissue at 27–28 h.p.i. (2 × 10 4 spores ml −1 in 0.25% gelatin solution) in 50 μg ml −1 BFA (0.1% DMSO). Treatments with the microtubule inhibitor methyl 1-(butylcarbamoyl)-2-benzimidazolecarbamate (MBC, the active ingredient in the fungicide benomyl) and the actin inhibitor LatA were performed on infected sheath tissue to examine the effects of hyphal cytoskeletal organization. Stock solutions of 10 mg ml −1 MBC (Sigma) and 100 μg ml −1 latrunculin A (Sigma) were prepared according to Czymmek et al . [47] . For in planta experiments with both drugs, we prepared working solutions of 50 μg ml −1 in 0.1% DMSO and treated the inoculated tissue as described for BFA. Fluorescence recovery after photobleaching Experiments were performed using a Zeiss LSM 510 confocal microscope with a 488-nm argon laser and a C-Apochromat × 40/1.2 NA water immersion objective at × 2 optical zoom. For FRAP analyses, the specific region of interest (ROI) covering the entire fluorescence in the BIC was selected for bleaching. We used 20 bleaching iterations at 100% laser power for a BIC containing cytoplasmic effector Pwl2:GFP fusion protein. Image scans were taken with the acousto-optic tunable filter attenuated to 5% laser power immediately before and after bleaching. Images were recorded up to 3 h after bleaching of the BIC region. During these time periods, the ROI showed from 70% to complete recovery. For quantitative analyses, the GFP fluorescence recovery curves were measured as the mean intensity of ROI pixels using the LSM software (version 4.2 SP1), normalized and graphed using Microsoft Excel. Vector construction and Agrobacterium-mediated transformation of M. oryzae Unless noted otherwise, transformation cassettes to observe M. oryzae fluorescently labelled cellular components and effector proteins were constructed containing the entire protein coding sequence with its native promoter (~1 kb) in a translational fusion with GFP, mRFP or mCherry. The GFP gene used was the EGFP gene from Clontech. The mRFP gene was obtained from Campbell et al . [48] . The mCherry gene from Shaner et al . [49] was isolated from pAN583. The plasmid containing the PWL2 promoter and coding sequence fused to a nuclear targeting mCherry:NLS sequence was obtained from Khang et al . [28] Each cassette was cloned into the pBHt2 binary vector for fungal transformation by A. tumefaciens [50] and for selection of positive transformants using resistance to hygromycin or geneticin (G418). Details of plasmid construction and corresponding fungal transformants used in this study are listed in Supplementary Tables S2 and S3 , respectively. M. oryzae field isolates O-137 (ref. 51 ) and Guy11 (ref. 52 ), and laboratory strain CP987 (ref. 51 ) were used as recipients. Fungal transformants were purified by isolation of single spores and 7–10 independent transformants were analysed per gene. In GenBank, the sequence data for the effector genes used in this study are under U26313 for PWL2, FJ807764 for Bas1, AF207841 for AVR-Pita1, MGG_10020.6 for Bas107, FJ807767 for Bas4, MGG_05785.6 for Bas113 and MGG_10097.6 for Slp1. Targeted gene replacements in M. oryzae and whole plant infection assays Targeted gene replacements for EXO70 , SEC5 and SSO1 were carried out using the split marker method [53] . A 1.4-kb hygromycin resistance cassette or a 2.8-kb sulphonylurea resistance cassette replaced the coding sequence of each gene. Sequence data for these genes can be found in the GenBank/EMBL databases under MGG_ numbers listed in Supplementary Table S1 . Sequences for flanking regions were retrieved from the M. oryzae genome database at the Broad Institute ( http://www.broadinstitute.org/annotation/fungi/magnaporthe/ ). Approximately 1.0 kb of flanking sequences were used for homologous recombination, and positive transformants were confirmed by DNA gel blot analysis ( Supplementary Fig. S5 ). At least two positive transformants were used for further analysis of every gene in each background. Whole plant infection assays for assessing mutant phenotypes were performed by spray inoculation of 2–3-week-old rice plants as described [41] . All results reported are based on at least three independent assays at each location. Generation of transgenic rice plants Gene fusions for expressing the plant plasma membrane marker low-temperature inducible protein 6B, LTi6B:GFP [54] and the ER marker GFP:HDEL [55] were transformed into rice cultivar Oryza sativa cv Sasanishiki [56] using standard rice transformation. Putative transformants of rice were selected on 100 μg ml −l hygromycin, confirmed by DNA gel blot, and expression checked by qRT–PCR, immunoblotting and epifluorescence microscopy. How to cite this article: Giraldo, M. C. et al . Two distinct secretion systems facilitate tissue invasion by the rice blast fungus Magnaporthe oryzae . Nat. Commun. 4:1996 doi: 10.1038/ncomms2996 (2013).